Transient activation of specific neurons in mice by selective expression of the capsaicin receptor The ability to control the electrical activity of a neuronal subtype is a valuable tool in deciphering the role of discreet cell populations in complex neural circuits. Recent techniques that allow remote control of neurons are either labor intensive and invasive or indirectly coupled to neural electrical potential with low temporal resolution. Here we show the rapid, reversible and direct activation of genetically identified neuronal subpopulations by generating two inducible transgenic mouse models. Confined expression of the capsaicin receptor, TRPV1, allows cell-specific activation after peripheral or oral delivery of ligand in freely moving mice. Capsaicin-induced activation of dopaminergic or serotonergic neurons reversibly alters both physiological and behavioural responses within minutes, and lasts ~10 min. These models showcase a robust and remotely controllable genetic tool that modulates a distinct cell population without the need for invasive and labour-intensive approaches. Understanding how complex neural circuits gather and process information to elicit behavioural responses is at the forefront of neuroscience. In this pursuit, it is useful to manipulate the biological characteristics of specific cell groups in a predictable manner. These alterations can be correlated to behavioural responses and used to draw conclusions about the role of the cell group in the neural circuit. Traditional tools, such as those involving pharmacological agents, electrical stimulation, and/or genetic manipulations have generated a wealth of information describing molecular correlates of many behaviours. However, many of these methods fall short with respect to temporal resolution or cellular specificity. Recent attempts to control neuronal signalling using genetically encoded effector proteins have allowed unprecedented access to electrical or molecular properties of cells [1] . Two techniques have been exceptionally useful in manipulating neural activity in freely moving animals. One of these, dubbed 'optogenetics', uses light-activated microbial opsins to modulate neural activity with millisecond precision [2] , [3] , [4] , [5] , [6] . However, the light delivery method required to activate these proteins is not only invasive, but also involves specialized equipment and is limited by tissue optical permeability. The other approach to regulate neural electrical activity is the use of engineered receptors that are activated by inert compounds which can penetrate the blood-brain barrier (BBB). Some of these 'designer receptors' do not necessitate invasive procedures (that is, cannula placement or viral vector delivery); however, their coarse kinetic resolution is not suitable for experiments that require rapid onset or recovery to baseline [1] , [7] , [8] , [9] , [10] , [11] . Given the respective limitations of these two approaches, a noninvasive method that could modulate genetically defined populations of neurons in a rapid reversible manner would fill a void in our current 'neural effector' tool set. Ectopic expression of the capsaicin-gated ion channel, TRPV1, which is most prominently expressed in the peripheral nervous system, has also been used successfully to activate neurons both in culture and in behaving animals [12] , [13] , [14] , [15] . This approach offers multiple advantages. TRPV1 is a non-selective cation channel that, when activated, depolarizes cells and rapidly induces action potentials in neurons [16] . Capsaicin, the pungent component of hot chili peppers, is a selective agonist of TRPV1 with a wide dynamic dose range [17] . In engineered mice, pan-neuronal TRPV1 expression has been used to drive neurons via unilateral striatal capsaicin infusion to evoke rotations that begin within seconds, and last for minutes [12] . Although this technique permits rapid reversible activation of neurons, it requires the delivery of capsaicin to the site of action via a cannula to avoid painful activation of peripheral TRPV1 receptors. To circumvent this problem, we generated mice that do not express TRPV1 from the endogenous locus but instead express TRPV1 solely in a genetically defined neuronal population. Here we demonstrate that systemic injection or voluntary consumption of capsaicin is sufficient to activate specific neural subtypes in these mice. When TRPV1 is selectively expressed in dopaminergic neurons, capsaicin administration increases the firing rate of this cell type leading to dopamine (DA) release within minutes. Varying doses of capsaicin modulate general activity and food consumption in freely moving mice. Furthermore, these mice develop a preference for capsaicin-containing water. On the other hand, high-dose capsaicin injection in mice, selectively expressing TRPV1 in serotonergic neurons, leads to hypolocomotion whereas lower doses evoke anxiogenic-like responses. Given its robust, rapid onset and offset coupled with its ease of use, this approach is a valuable addition to our existing neuromodulatory tools. Exclusive expression of TRPV1 in dopaminergic neurons Proper DA signalling accommodates a wide range of actions and lends itself to molecular manipulations that result in readily observable behaviours [18] , [19] . To test the plausibility of exogenous TRPV1-dependent activation of a genetically identified subpopulation of neurons in vivo , we generated mice that express the capsaicin receptor exclusively in the dopaminergic neurons by utilizing a triple transgenic approach (DAT–TRPV1; Fig. 1a ). To avoid painful activation of peripheral TRPV1-containing neurons, DAT–TRPV1 and control lines, Slc6a3 Cre (DAT-Cre) or Gt(ROSA)26Sor-stop flox -Trpv1-ires-ECFP (R26-TRPV1) were generated on Trpv1 knockout background [12] , [17] , [20] . We tested specific functional expression of the rat Trpv1 transgene in dopaminergic neurons by intraperitoneal (i.p.) injections of capsaicin followed by double immunofluorescence labelling of c-Fos, a neural activity marker, and tyrosine hydroxylase (TH), the rate-limiting enzyme in DA synthesis. In the midbrain of capsaicin-injected DAT–TRPV1 mice, 96.2±0.7% of the cells that were TH immunoreactive were also positive for c-Fos (compared with 4.8±2.1% of TH cells in vehicle-injected mice; Student's t -test: P <0.001; Fig. 1b ). Neither of the capsaicin-injected control lines demonstrated significant c-Fos immunoreactivity in midbrain TH-positive cells ( Supplementary Fig. S1a-c ). Pharmacologically induced DA release and DA D1 receptor agonists increase immediate early gene expression in brain regions innervated by dopaminergic neurons [21] , [22] , [23] . In accordance with capsaicin-induced activation of DA neurons and neurotransmitter release, we detected an elevated number of c-Fos-immunoreactive cells within most DA targets in capsaicin-injected DAT–TRPV1 mice but not controls ( Fig. 1c,d ; Supplementary Fig. S1d-o ). Although there was no appreciable increase in the number of c-Fos-immunoreactive hippocampal cells in capsaicin-injected DAT–TRPV1 mice, we observed an increase in the lateral habenula and piriform cortex compared with vehicle-injected DAT–TRPV1 mice ( Supplementary Fig. S2a-f ). These results indicate that capsaicin increases activity-dependent gene expression in DA neurons and their targets in DAT–TRPV1 mice. 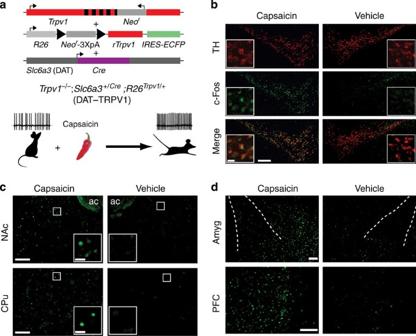Figure 1: Capsaicin receptor is selectively expressed in dopaminergic neurons. (a) Triple transgenic mice conditionally express ratTrpv1(rTrpv1) gene fromGt(ROSA)26Sor(R26) locus only in Cre recombinase producing neurons under the control of DA transporter (Slc6a3or DAT) promoter on theTrpv1knockout background (DAT–TRPV1;Neor: neomycin resistance gene; IRES-ECFP: internal ribosome entry site-enhanced cyan fluorescent protein). The specific excision of theloxP-flanked transcriptional termination cassette only in DAT-expressing cells allows expression of the capsaicin receptor exclusively in the dopaminergic cells. After capsaicin administration, neural firing is expected to increase only in TRPV1- expressing cells and lead to behavioural consequences. (b) Double-fluorescent immunohistochemistry with TH (top) and c-Fos (middle) antibody of midbrain 90 min after capsaicin (32 mg kg−1; left) or vehicle (right) injection in DAT–TRPV1 mice (n=4 for each group). Pseudo-coloured images (TH: red and cFos: green) are merged at the bottom panel. Scale bar, 200 μm, inset scale bar 20 μm. (c,d) Fluorescent immunohistochemistry with c-Fos antibody of dopaminergic innervation targets 90 min after capsaicin (32 mg kg−1; left) or vehicle (right) injection in DAT–TRPV1 mice (NAc: nucleus accumbens; CPu: caudate putamen; Amyg: amygdala; PFC: prefrontal cortex; ac: anterior commissure;n=3–4 per group). Scale bar, 100 μm. Insets are zoomed images of indicated areas in (c); scale bars, 20 μm. Figure 1: Capsaicin receptor is selectively expressed in dopaminergic neurons. ( a ) Triple transgenic mice conditionally express rat Trpv1 ( rTrpv1 ) gene from Gt(ROSA)26Sor (R26) locus only in Cre recombinase producing neurons under the control of DA transporter ( Slc6a3 or DAT) promoter on the Trpv1 knockout background (DAT–TRPV1; Neo r : neomycin resistance gene; IRES-ECFP: internal ribosome entry site-enhanced cyan fluorescent protein). The specific excision of the loxP -flanked transcriptional termination cassette only in DAT-expressing cells allows expression of the capsaicin receptor exclusively in the dopaminergic cells. After capsaicin administration, neural firing is expected to increase only in TRPV1- expressing cells and lead to behavioural consequences. ( b ) Double-fluorescent immunohistochemistry with TH (top) and c-Fos (middle) antibody of midbrain 90 min after capsaicin (32 mg kg −1 ; left) or vehicle (right) injection in DAT–TRPV1 mice ( n =4 for each group). Pseudo-coloured images (TH: red and cFos: green) are merged at the bottom panel. Scale bar, 200 μm, inset scale bar 20 μm. ( c , d ) Fluorescent immunohistochemistry with c-Fos antibody of dopaminergic innervation targets 90 min after capsaicin (32 mg kg −1 ; left) or vehicle (right) injection in DAT–TRPV1 mice (NAc: nucleus accumbens; CPu: caudate putamen; Amyg: amygdala; PFC: prefrontal cortex; ac: anterior commissure; n =3–4 per group). Scale bar, 100 μm. Insets are zoomed images of indicated areas in ( c ); scale bars, 20 μm. Full size image Capsaicin-induced TRPV1 activation and subsequent calcium influx can cause cell death in some cell types [12] . However, 24 h after i.p. capsaicin administration, we did not observe any microglial activation, an early indicator of neuronal damage, in DAT–TRPV1 or control mice ( Fig. 2a ) [24] . Furthermore, even after 10 capsaicin injections over a 30-day period, there was no obvious reduction in TH-immunoreactive neurons in the ventral tegmental area/substantia nigra pars compacta (VTA/SNc) or in the intensity of TH staining in the striatum of capsaicin-injected DAT–TRPV1 mice compared with controls ( Fig. 2b ). 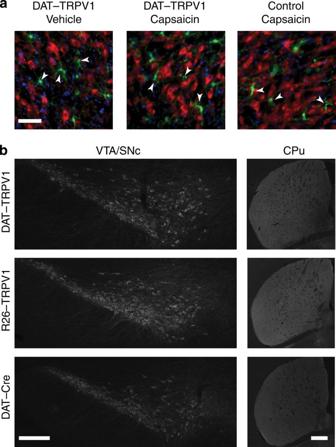Figure 2: Capsaicin administration does not induce apparent cell death in DAT–TRPV1 mice. (a) Pseudo-coloured images of fluorescent immunohistochemistry with TH (red), ionized calcium-binding molecule-1 (Iba-1, a marker for microglial cells; green) antibody and DAPI (blue) staining 24 h after capsaicin (32 mg kg−1) or vehicle administration. Microglia (arrowheads) remain ramified in the midbrain of DAT–TRPV1 mice following capsaicin administration implicating normal homeostasis and lack of neuropathology. Scale bar, 50 μm. (b) Following 10 i.p. injections of capsaicin (32 mg kg−1) through 30-day period, TH fluorescent immunohistochemistry of VTA/SNc and CPu of DAT–TRPV1, R26-TRPV1 or DAT-Cre mice (n=3–4 per group). Only a single dose of capsaicin was administered per day. Scale bars, 200 μm. Figure 2: Capsaicin administration does not induce apparent cell death in DAT–TRPV1 mice. ( a ) Pseudo-coloured images of fluorescent immunohistochemistry with TH (red), ionized calcium-binding molecule-1 (Iba-1, a marker for microglial cells; green) antibody and DAPI (blue) staining 24 h after capsaicin (32 mg kg −1 ) or vehicle administration. Microglia (arrowheads) remain ramified in the midbrain of DAT–TRPV1 mice following capsaicin administration implicating normal homeostasis and lack of neuropathology. Scale bar, 50 μm. ( b ) Following 10 i.p. injections of capsaicin (32 mg kg −1 ) through 30-day period, TH fluorescent immunohistochemistry of VTA/SNc and CPu of DAT–TRPV1, R26-TRPV1 or DAT-Cre mice ( n =3–4 per group). Only a single dose of capsaicin was administered per day. Scale bars, 200 μm. Full size image Capsaicin-dependent activation and DA release To confirm that capsaicin administration leads to activation of dopaminergic cells in DAT–TRPV1 mice, we performed whole-cell, voltage-clamp recordings from midbrain slices. The amount of current required to clamp dopaminergic cells at −70 mV did not differ between groups (control: −112.5±19.4 pA versus DAT–TRPV1: −137.5±20.2 pA; n =11–12; Student's t -test: P =0.38). A high concentration of capsaicin induced large inward currents within minutes that lasted ~15 min ( Fig. 3a ), similar to capsaicin-induced endogenous TRPV1 currents reported in dorsal root ganglia [25] . Although the baseline firing rates of dopaminergic neurons were similar between the two groups (control: 0.84±0.11 Hz versus DAT–TRPV1: 0.82±0.14 Hz; n =10–12; Student's t -test: P =0.91), a moderate concentration of capsaicin (0.1 μM) was sufficient to increase the spiking activity of DA neurons from DAT–TRPV1 mice but not controls ( Fig. 3b,c ). Surprisingly, action potentials were completely inhibited in six out of eight cells recorded with the two highest doses of capsaicin application. This is presumably due to the depolarization-induced inactivation of voltage-gated sodium channels, a phenomenon that has been previously observed [15] . These data demonstrate that TRPV1 is functionally expressed in dopaminergic cells in DAT–TRPV1 mice, but not in controls, and capsaicin administration induces inward currents thereby increasing neuronal activity. 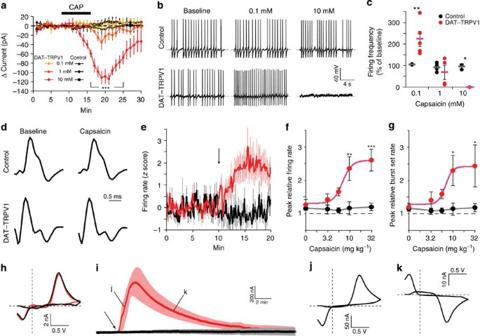Figure 3: Capsaicin increases neural activity and induces DA release in DAT–TRPV1 mice. (a–c) DA neuron whole-cell electrophysiology in midbrain explants of DAT–TRPV1 mice. (a) Voltage-clamp recordings after capsaicin application. 10 μM dose induced significantly larger currents in neurons from DAT–TRPV1 mice (n=11–12, two-way repeated measures ANOVA: group×time effect,F(70,280)=4.24,P<0.0001). (b) Sample traces of current-clamp recordings from a single DAT–TRPV1 (top) or control (bottom) neuron before (left), during 0.1 μM (middle) or 10 μM (right) capsaicin application. (c) Summary of capsaicin-induced change in firing rate from (b) normalized to baseline (n=3–5, two-way ANOVA: genotype×dose effect,F(2,17)=9.94,P=0.0014, Bonferroni post test,P<0.01. Horizontal grey (control) or pink (DAT–TRPV1) bars indicate mean. (d–g) Single-unit recordings from putative DA neurons in awake and freely moving DAT–TRPV1 mice. (d) Sample traces of putative DA neuron single-unit waveforms before and after capsaicin (10 mg kg−1) administration in control and DAT–TRPV1 mice. (e) Single-unit firing rate standard-score (zscore) from DA neurons after capsaicin administration (10 mg kg−1i.p.; arrow) from control (black,n=7) and DAT–TRPV1 (red,n=16) mice. (f) Dose-response profile of maximum firing rate of single units after capsaicin administration from control (black with grey fitted curve; EC50: 7.2 mg kg−1(LogEC50=0.86±0.11); Hill coefficient: 3.9;n=7–21) or DAT–TRPV1 (red with pink fitted curve,n=9–18) mice (two-way ANOVA: genotype×dose effect,F(4,121)=3.58,P=0.0085). (g) Dose-response profile of maximum burst set rate of single units after capsaicin administration from control (black) or DAT–TRPV1 (red; EC50: 6.9 mg kg−1(LogEC50=0.84±0.15); Hill coefficient=4.8) mice (two-way ANOVA: genotype effect,F(1,121)=13.88,P=0.0003). (h–k) Cyclic voltammetry recordings in anaesthetized DAT–TRPV1 mice. (h) Electrical stimulation induced representative cyclic voltammograms from control (black) and DAT–TRPV1 (red) mice. Peak oxidation currents were not significantly different between the two groups (controlsn=3, 3.7±1.2 nA; DAT–TRPV1n=5, 5.9±1.4 nA). (i) Averaged DA oxidation currents in response to capsaicin administration (32 mg kg−1i.p.) in control (black) or DAT–TRPV1 (red) mice (arrow indicates initial detectable DA signal). (j,k) Representative background subtracted cyclic voltammograms during the ascending (j) and descending (k) phase of capsaicin-induced response at indicated time points in (i). Error bars±s.e.m. Bonferroni post tests, *P<0.05, **P<0.01, ***P<0.001. Figure 3: Capsaicin increases neural activity and induces DA release in DAT–TRPV1 mice. ( a – c ) DA neuron whole-cell electrophysiology in midbrain explants of DAT–TRPV1 mice. ( a ) Voltage-clamp recordings after capsaicin application. 10 μM dose induced significantly larger currents in neurons from DAT–TRPV1 mice ( n =11–12, two-way repeated measures ANOVA: group×time effect, F (70,280) =4.24, P <0.0001). ( b ) Sample traces of current-clamp recordings from a single DAT–TRPV1 (top) or control (bottom) neuron before (left), during 0.1 μM (middle) or 10 μM (right) capsaicin application. ( c ) Summary of capsaicin-induced change in firing rate from ( b ) normalized to baseline ( n =3–5, two-way ANOVA: genotype×dose effect, F (2,17) =9.94, P =0.0014, Bonferroni post test, P <0.01. Horizontal grey (control) or pink (DAT–TRPV1) bars indicate mean. ( d – g ) Single-unit recordings from putative DA neurons in awake and freely moving DAT–TRPV1 mice. ( d ) Sample traces of putative DA neuron single-unit waveforms before and after capsaicin (10 mg kg −1 ) administration in control and DAT–TRPV1 mice. ( e ) Single-unit firing rate standard-score ( z score) from DA neurons after capsaicin administration (10 mg kg −1 i.p. ; arrow) from control (black, n =7) and DAT–TRPV1 (red, n =16) mice. ( f ) Dose-response profile of maximum firing rate of single units after capsaicin administration from control (black with grey fitted curve; EC 50 : 7.2 mg kg −1 (LogEC 50 =0.86±0.11); Hill coefficient: 3.9; n =7–21) or DAT–TRPV1 (red with pink fitted curve, n =9–18) mice (two-way ANOVA: genotype×dose effect, F (4,121) =3.58, P =0.0085). ( g ) Dose-response profile of maximum burst set rate of single units after capsaicin administration from control (black) or DAT–TRPV1 (red; EC 50 : 6.9 mg kg −1 (LogEC 50 =0.84±0.15); Hill coefficient=4.8) mice (two-way ANOVA: genotype effect, F (1,121) =13.88, P =0.0003). ( h – k ) Cyclic voltammetry recordings in anaesthetized DAT–TRPV1 mice. ( h ) Electrical stimulation induced representative cyclic voltammograms from control (black) and DAT–TRPV1 (red) mice. Peak oxidation currents were not significantly different between the two groups (controls n =3, 3.7±1.2 nA; DAT–TRPV1 n =5, 5.9±1.4 nA). ( i ) Averaged DA oxidation currents in response to capsaicin administration (32 mg kg −1 i.p.) in control (black) or DAT–TRPV1 (red) mice (arrow indicates initial detectable DA signal). ( j , k ) Representative background subtracted cyclic voltammograms during the ascending ( j ) and descending ( k ) phase of capsaicin-induced response at indicated time points in ( i ). Error bars±s.e.m. Bonferroni post tests, * P <0.05, ** P <0.01, *** P <0.001. Full size image To test the electrophysiological properties of capsaicin-activated neurons in awake and freely moving animals, we chronically implanted DAT–TRPV1 ( n =8) and control ( n =4) mice with recording electrodes in the VTA/SNc. We identified 131 putative DA neurons based on waveform dynamics, firing pattern criteria and tetrode placement ( Supplementary Fig. S3 ). After 10 min of baseline recording (baseline firing rate control: 6.23±0.53 Hz versus DAT–TRPV1: 5.65±0.54 Hz; n =59–72; Student's t -test: P =0.44), mice were injected with varying doses of capsaicin or vehicle. DAT–TRPV1 and control putative DA neuron action potential waveforms were similar and did not show appreciable changes in their kinetics after capsaicin injections ( Fig. 3d ). As expected, capsaicin injections increased the firing rate of putative DA neurons of DAT–TRPV1 mice within 2 min whereas firing rate of neurons from control mice did not change ( Fig. 3e ). Both peak firing rate and burst activity of putative DA neurons from DAT–TRPV1 mice increased dose-dependently indicating that capsaicin is capable of augmenting dopaminergic neural activity in freely moving DAT–TRPV1 mice ( Fig. 3f,g ). We utilized fast-scan cyclic voltammetry (FSCV) in anaesthetized mice to determine whether capsaicin-induced increases in neural activity enhances DA release. First, we confirmed that direct stimulation of DA neuron fibres in the medial forebrain bundle (MFB) evoked DA release similarly in both control and DAT–TRPV1 mice ( Fig. 3h ). Subsequently, we administered capsaicin (32 mg kg −1 , i.p.) after 2 min of baseline recording. Within 3.8±1.5 min of drug administration, DA release was evident in DAT–TRPV1 but not in control mice ( Fig. 3i ). This response peaked within 3 min and returned to baseline after 20 min. Background-subtracted cyclic voltammograms confirmed that the ascending and descending phase of the response corresponded to the increasing and decreasing levels of released DA, respectively ( Fig. 3j,k ). Taken together, these results indicate that capsaicin-evoked inward currents increase neural activity and DA release in DAT–TRPV1 mice. Capsaicin-induced behavioural responses in DAT–TRPV1 mice Elevation in DA levels in the striatum facilitates movement via both the direct and indirect pathways and increases general locomotor activity [26] . To test whether the capsaicin-induced increase in dopaminergic neural activity is able to influence locomotor behaviour, we video-recorded mice after injections of vehicle or varying doses of capsaicin. When introduced to a novel environment after vehicle injection, DAT–TRPV1 and control mice explored the arena in a similar manner ( Supplementary Movie 1 ). Following ~2 h of habituation, capsaicin administration elevated the activity of only the DAT–TRPV1 mice ( Supplementary Movie 2 ). Treatment with the two highest doses of capsaicin (10 and 32 mg kg −1 bodyweight) evoked the most evident responses within minutes. This capsaicin-induced locomotor response returned to control levels 15 min after drug administration ( Supplementary Movie 3 ). To assess the reproducibility of capsaicin-induced locomotion in DAT–TRPV1 mice, we administered capsaicin to mice once a day for 5 consecutive days and video-recorded their activity. Within 10 min of receiving capsaicin at 10 mg kg −1 , DAT–TRPV1 mice showed elevated locomotion each day ( Supplementary Fig. S4a ). Surprisingly, animals injected with capsaicin at 32 mg kg −1 on the first few days travelled less distance than mice injected with 10 mg kg −1 , but, by day 4, their responses were similar to each other. This apparent behavioural sensitization is similar to the increased locomotor activity elicited by repeated administration of psychostimulants that release DA [27] . This was most evident when comparing the dose-response profiles of distance travelled between days 1 and 5 of capsaicin injections ( Fig. 4a ). The lower activity during days 1 through 3 for capsaicin injection at 32 mg per kg body weight is a reflection of some DAT–TRPV1 mice 'freezing' for short durations during the heightened activity period generating an inverted-U shaped dose-response profile akin to dose-response profiles of some psychostimulants ( Supplementary Movie 2 , red arrowhead) [28] . Capsaicin-induced hyperactivity returned to baseline after 10 min at all doses ( Supplementary Fig. S4b ). To uncover the temporal dynamics of the locomotor response in finer detail, we measured the number of beam breaks made by capsaicin- (10 mg kg −1 ) or vehicle-injected DAT–TRPV1 or control mice ( Fig. 4b ). Following the capsaicin injection, DAT–TRPV1 mice had elevated activity within ~2.5 min that peaked at ~8 min and lasted for ~11.5 min. Therefore, capsaicin-induced neural activation can elicit reversible, dose-dependent behavioural responses. 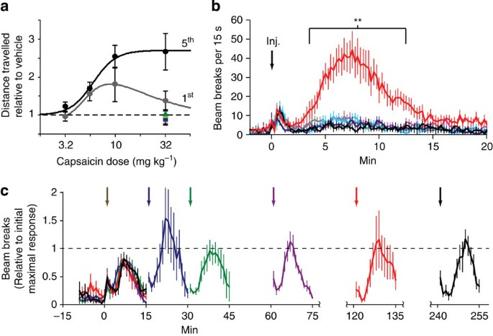Figure 4: Capsaicin-induced locomotion in DAT–TRPV1 mice. (a) Dose-response curves comparing distance travelled during first day (grey) to the fifth day (black) of DAT–TRPV1 capsaicin injections (n=7–10 per group; First day bell-shape curve, peak value: 9.1 mg kg−1versus fifth day sigmoidal curve, EC50=6.0 mg kg−1, Hill coefficient: 3.8). Capsaicin (32 mg kg−1)-induced responses of R26-TRPV1 (green triangles) and DAT-Cre (blue squares) control mice during first (lighter) and last (darker) day. (b) Beam breaks per 15 s made by control (R26-TRPV1: black; DAT-Cre: blue) or DAT–TRPV1 (red) mice after vehicle (lighter) or capsaicin administration (darker; 10 mg kg−1; inj.: time of injection;n=9–12 per group; two-way repeated measures ANOVA: group×time effect,F(1215,13122)=5.33,P<0.0001; Bonferroni post test, **P<0.01). (c) Activity response of DAT–TRPV1 mice to two capsaicin injections (5.6 mg kg−1) separated by 15 (blue), 30 (green), 60 (purple), 120 (red) or 240 (black) min (n=6 per group). Capsaicin-induced activity per minute is normalized to the peak during the initial capsaicin response (brown arrow indicates time of first injection). For simplicity, only 15 min after the second capsaicin injection (arrows) is plotted. Note gaps in time axis. Figure 4: Capsaicin-induced locomotion in DAT–TRPV1 mice. ( a ) Dose-response curves comparing distance travelled during first day (grey) to the fifth day (black) of DAT–TRPV1 capsaicin injections ( n =7–10 per group; First day bell-shape curve, peak value: 9.1 mg kg −1 versus fifth day sigmoidal curve, EC 50 =6.0 mg kg −1 , Hill coefficient: 3.8). Capsaicin (32 mg kg −1 )-induced responses of R26-TRPV1 (green triangles) and DAT-Cre (blue squares) control mice during first (lighter) and last (darker) day. ( b ) Beam breaks per 15 s made by control (R26-TRPV1: black; DAT-Cre: blue) or DAT–TRPV1 (red) mice after vehicle (lighter) or capsaicin administration (darker; 10 mg kg −1 ; inj. : time of injection; n =9–12 per group; two-way repeated measures ANOVA: group×time effect, F (1215,13122) =5.33, P <0.0001; Bonferroni post test, ** P <0.01). ( c ) Activity response of DAT–TRPV1 mice to two capsaicin injections (5.6 mg kg −1 ) separated by 15 (blue), 30 (green), 60 (purple), 120 (red) or 240 (black) min ( n =6 per group). Capsaicin-induced activity per minute is normalized to the peak during the initial capsaicin response (brown arrow indicates time of first injection). For simplicity, only 15 min after the second capsaicin injection (arrows) is plotted. Note gaps in time axis. Full size image In certain conditions, prolonged capsaicin administration has been demonstrated to desensitize TRPV1 to a subsequent application [29] . Similar acute desensitization might underlie the mechanism of rapid offset of capsaicin-induced responses in DAT–TRPV1 mice. To test this possibility, we measured activity after two capsaicin injections separated by 15, 30, 60, 120 or 240 min. As expected, DAT–TRPV1 mice had a marked increase in activity after 5.6 mg per kg capsaicin administration ( Supplementary Fig. S4c ). Compared with this initial response, subsequent capsaicin injections induced similar levels of heightened activity regardless of time separation ( Fig. 4c ). This result argues against desensitization of TRPV1 as the mechanism for fast reversal of behavioural responses and demonstrates the plausibility of repeated activation in rapid succession. The role of DA in goal-directed behaviours is well established [19] . To test the ability of capsaicin-induced neural activation to influence the ability of mice to work for food, we trained mice to press a lever for food pellets. We then tested whether varying doses of capsaicin administration would modulate responses in a daily progressive-ratio (PR) task. Within 15 min of drug administration, the two highest doses of capsaicin inhibited lever pressing and food-hopper head-entry rates of DAT–TRPV1 mice without affecting non-contingent (nose-poke) responses during the PR session ( Supplementary Fig. S5a,b ). This inhibition returned to baseline within the last 15 min of the 60-min session ( Supplementary Fig. S5c,d ). At high doses, drugs that enhance or mimic DA can suppress incentive for food similar to the capsaicin-induced responses observed here [30] , [31] , [32] . However, at lower doses these pharmacological agents can induce increased motivation for food similar to some mouse models with hyperdopaminergia [33] , [34] , [35] . Surprisingly, lower doses of capsaicin (3.2 and 5.6 mg kg −1 ) that elicit neural activation did not affect the behaviour of DAT–TRPV1 mice in the PR task. It is possible that overtrained mice in operant conditioning chambers confounded our ability to observe more subtle differences. Therefore, we tested whether capsaicin could modulate free-access feeding in DAT–TRPV1 mice at these doses. To engage mice in feeding during the effective period of capsaicin administration, we fasted mice for 22 h and determined their latency to feed following vehicle or capsaicin (5.6 mg kg −1 i.p.) injections. DAT–TRPV1 mice injected with capsaicin began food consumption ~3.5 min after control mice injected with capsaicin or DAT–TRPV1 mice injected with vehicle ( Fig. 5a ). Interestingly, although slower to commence feeding, DAT–TRPV1 capsaicin-injected mice became hyperphagic and consumed the same amount of food as control mice by 18 min of free-food access ( Fig. 5b ). To circumvent the initial hypophagic phase, we tested whether a lower dose of capsaicin (3.2 mg kg −1 ) could decrease the latency to begin feeding after 14 h of food restriction. The shorter duration of fasting increased the latency of control mice to commence feeding ( Fig. 5c ). Under these conditions, capsaicin-administered to DAT–TRPV1 mice initiated feeding ~4.5 min faster than controls ( Fig. 5c,d ). These findings suggest that activation of dopaminergic neurons can either enhance or inhibit feeding. 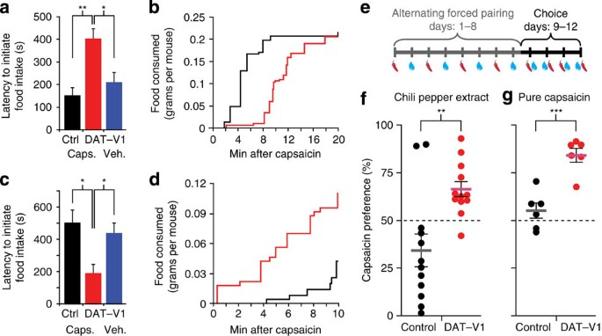Figure 5: Capsaicin-induced behavioural responses in DAT–TRPV1 mice. (a) Latency to initiate feeding by vehicle or capsaicin (5.6 mg kg−1) administered to DAT–TRPV1 or control mice after 22 h of fasting (n=5–10; one-way ANOVA,F(2,17)=8.38,P=0.0029; Tukey's multiple comparison post tests: *P<0.05, **P<0.01). (b) Amount of food consumed over time by capsaicin-injected DAT–TRPV1 (red) or control (black) mice in (a). (c) Latency to initiate feeding by vehicle or capsaicin (3.2 mg kg−1) administered to DAT–TRPV1 or control mice after 14 h of fasting (n=5–6; one-way ANOVA,F(2,14)=6.22,P=0.0117; Tukey's multiple comparison post tests: *P<0.05). (d) Amount of food consumed over time by capsaicin injected DAT–TRPV1 (red) or control (black) mice in (c). (e) Schematic demonstration of two-bottle preference test. Mice were allowed to drink either water with vehicle or water containing hot chili pepper extract on alternating days during the initial 8 days and given a choice during days 9–12. (f) Percent preference of control (black) or DAT–TRPV1 (red) mice for hot chili pepper extract (n=12 per group). (g) Percent preference for pure capsaicin (n=6 per group). Horizontal grey (control) or pink (DAT–TRPV1) bars indicate mean. Student'st-test **P<0.01, ***P<0.001. Error bars±s.e.m. Caps.: capsaicin; Veh.: Vehicle. Figure 5: Capsaicin-induced behavioural responses in DAT–TRPV1 mice. ( a ) Latency to initiate feeding by vehicle or capsaicin (5.6 mg kg −1 ) administered to DAT–TRPV1 or control mice after 22 h of fasting ( n =5–10; one-way ANOVA, F (2,17) =8.38, P =0.0029; Tukey's multiple comparison post tests: * P <0.05, ** P <0.01). ( b ) Amount of food consumed over time by capsaicin-injected DAT–TRPV1 (red) or control (black) mice in ( a ). ( c ) Latency to initiate feeding by vehicle or capsaicin (3.2 mg kg −1 ) administered to DAT–TRPV1 or control mice after 14 h of fasting ( n =5–6; one-way ANOVA, F (2,14) =6.22, P =0.0117; Tukey's multiple comparison post tests: * P <0.05). ( d ) Amount of food consumed over time by capsaicin injected DAT–TRPV1 (red) or control (black) mice in ( c ). ( e ) Schematic demonstration of two-bottle preference test. Mice were allowed to drink either water with vehicle or water containing hot chili pepper extract on alternating days during the initial 8 days and given a choice during days 9–12. ( f ) Percent preference of control (black) or DAT–TRPV1 (red) mice for hot chili pepper extract ( n =12 per group). ( g ) Percent preference for pure capsaicin ( n =6 per group). Horizontal grey (control) or pink (DAT–TRPV1) bars indicate mean. Student's t -test ** P <0.01, *** P <0.001. Error bars±s.e.m. Caps. : capsaicin; Veh. : Vehicle. Full size image A variety of lesion, stimulation and pharmacological techniques have demonstrated that activation of DA neurons and consequent DA release is a neural substrate encoding reward [19] . We assessed whether capsaicin-induced activation of DA neurons in DAT–TRPV1 mice alters the incentive value of capsaicin in a two-bottle preference test. After alternating presentations of hot chili pepper extract or vehicle during the 8 forced-choice days, mice were allowed to choose between the two water bottles freely for 4 days ( Fig. 5e ). Although wild-type mice (expressing endogenous TRPV1) do not drink capsaicin-containing water, TRPV1 knockout mice consume capsaicin-treated water without any obvious adverse effects [17] . On the first forced-choice day of capsaicin-spiked water, DAT–TRPV1 and control mice consumed similar amounts of solution. Within 30-min bins, DAT–TRPV1 mice drank on average 0.19±0.01 ml of capsaicin solution during the highest consumption period (ZT 14–18). This amount of capsaicin, if administered i.p., is within the dynamic range of capsaicin-induced physiological and behavioural responses described above. When given a choice between bottles, 11 out of 12 DAT–TRPV1 mice preferred capsaicin-containing solution ( Fig. 5f ). Interestingly, 10 out of 12 control mice showed aversion to the capsaicin-containing water, possibly because of TRPV1-independent detection of unpalatable components in the hot chili pepper extract. Therefore, we performed a two-bottle preference test with pure capsaicin, instead of hot chili pepper extract. In this assay, control mice had no preference for either bottle while DAT–TRPV1 mice demonstrated strong preference for capsaicin-containing solution ( Fig. 5g ) confirming the presence of aversive compounds in hot chili pepper extract. These results emphasize that elevated dopaminergic activity, associated with capsaicin consumption, is sufficient for it to acquire incentive value in DAT–TRPV1 mice. Activation of serotonergic neurons by capsaicin To demonstrate the translatability of this technique to other neural systems, we applied a similar strategy to serotonergic neurons. We bred R26-TRPV1 mice with BAC transgenics expressing Cre recombinase under the control enhancer region of the Pet1 gene (ePet–Cre). The expression of this transgene is restricted to serotonin (5-HT) neurons [36] . As with DAT–TRPV1 mice, to circumvent peripheral TRPV1 activation, all lines were generated on the Trpv1 knockout background [17] . Therefore, in this triple transgenic model, the excision of the upstream loxP -flanked transcriptional termination cassette from the Gt(ROSA)26Sor locus allows the expression of the rat Trpv1 transgene only in serotonergic neurons (ePet–TRPV1). To test for functional TRPV1 expression in serotonergic cells, we systemically administered capsaicin (32 mg kg −1 ) or vehicle to ePet–TRPV1 or control mice and performed double immunohistochemistry for the neural activity marker c-Fos and tryptophan hydroxylase (TPH), an enzyme essential for 5-HT synthesis. In ePet–TRPV1 mice injected with capsaicin, 71.2±3.4% of TPH-immunostained neurons were also c-Fos positive compared with 10.5±3.8% in mice injected with vehicle ( n =3 per group, Student's t -test: P <0.001, Fig. 6a ). R26-TRPV1 and ePet–Cre control mice injected with capsaicin had similar percentage of co-staining to vehicle-injected ePet–TRPV1 animals ( Supplementary Fig. S6 ). This result implicates functional expression of TRPV1 channel in serotonergic neurons of ePet–TRPV1 mice. 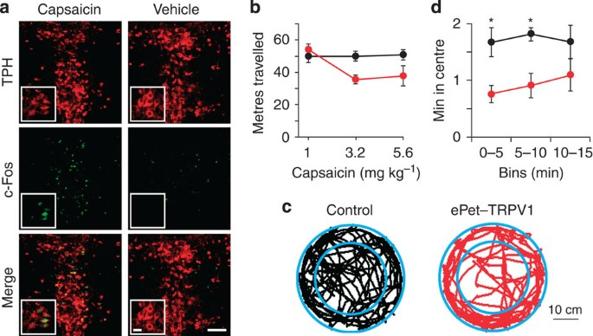Figure 6: Capsaicin-induced responses in ePet–TRPV1 mice. (a) Double-fluorescent immunohistochemistry with TPH (top) and c-Fos (middle) antibody in the dorsal raphe 90 min after capsaicin (32 mg kg−1; left) or vehicle (right) injection of ePet–TRPV1 mice. Pseudo-coloured images (TPH: red and cFos: green) are merged at the bottom panel. Scale bar, 100 μm, inset scale bar 20 μm. (b) Distance travelled within 15 min by control (black) or ePet–TRPV1 (red) mice in an open-field after indicated doses of capsaicin administration (n=6–8). (c) Initial 5-min sample path traces in an open-field of control (black) or ePet–TRPV1 (red) mice following capsaicin injection (1 mg kg−1). (d) Time spent in the centre from (c) in 5-min bins (black: control; red: ePet–TRPV1; two-way repeated measures ANOVA: genotype effectF(1,12)=10.01,P=0.0082). Error bars±s.e.m. Bonferroni post tests, *P<0.05. Figure 6: Capsaicin-induced responses in ePet–TRPV1 mice. ( a ) Double-fluorescent immunohistochemistry with TPH (top) and c-Fos (middle) antibody in the dorsal raphe 90 min after capsaicin (32 mg kg −1 ; left) or vehicle (right) injection of ePet–TRPV1 mice. Pseudo-coloured images (TPH: red and cFos: green) are merged at the bottom panel. Scale bar, 100 μm, inset scale bar 20 μm. ( b ) Distance travelled within 15 min by control (black) or ePet–TRPV1 (red) mice in an open-field after indicated doses of capsaicin administration ( n =6–8). ( c ) Initial 5-min sample path traces in an open-field of control (black) or ePet–TRPV1 (red) mice following capsaicin injection (1 mg kg −1 ). ( d ) Time spent in the centre from ( c ) in 5-min bins (black: control; red: ePet–TRPV1; two-way repeated measures ANOVA: genotype effect F (1,12) =10.01, P =0.0082). Error bars±s.e.m. Bonferroni post tests, * P <0.05. Full size image We investigated whether TRPV1-induced activation of serotonergic neurons had behavioural consequences. Increases in brain 5-HT has been demonstrated to affect anxiety-related behaviours [37] . Therefore, we video-recorded ePet–TRPV1 and control mice in an open-field, following administration of capsaicin. Interestingly, doses that are below the EC 50 of behavioural and physiological responses in DAT–TRPV1 model (3.2 and 5.6 mg kg −1 ) induced hypolocomotion in ePet–TRPV1 mice ( Fig. 6b ). This response is similar to mice that have been administered some 5-HT receptor agonists [38] . Because changes in locomotive behaviour of mice could interfere with proper analysis in the open-field test, we used capsaicin at a dose (1 mg kg −1 ) that did not have adverse effects on mouse activity level. Similar to the acute axiogenic-like effects of some drugs that elevate extracellular 5-HT levels, this dose of capsaicin-induced thigmotaxis during the 15-min session ( Fig. 6c ; time spent around the edges: control, n =8, 9.8±0.5 min; ePet–TRPV1, n =6, 12.2±0.6 s; Student's t -test P <0.05) [39] , [40] . To gain further insight to the temporal resolution of this response, we analysed each 5-min bin and determined the time spent by mice in the centre of the field. During the initial two bins, ePet–TRPV1 mice explored the centre of the field less than control mice, an effect that was alleviated during the last 5 min of the session ( Fig. 6d ). Therefore, similar to DAT–TRPV1 mice, capsaicin-induced serotonergic activity and the subsequent behavioural response had a rapid onset and lasted for ~10 min. We developed a conditional transgenic mouse model that rapidly and reversibly elevates neural activity of a genetically defined population of neurons without requiring invasive techniques. The selective TRPV1 expression-mediated activation (STEMA) of neurons allows for fast activity onset and subsequent behavioural responses that depend on the specified neural type. Contrary to previous speculations, the potent TRPV1 ligand capsaicin is able to cross the BBB and can be delivered orally or via systemic injections [1] . TRPV1-induced neural activity peaks within 7 min, lasts for only ~10 min, and can be repeated immediately. We applied STEMA to stimulate dopaminergic or serotonergic neurons in freely moving mice and report physiological and behavioural responses that underline not only its ease of use but also its effectiveness in modulating neural subtypes (see Supplementary Discussion for a detailed discussion of capsaicin-induced DAT–TRPV1 and ePet–TRPV1 behavioural phenotypes). In recent years, there have been great advancements in the ability to reversibly and bidirectionally modulate neural activity in behaving rodents with genetically encoded effector proteins [1] , [5] , [41] . Two techniques that increase neural firing have been especially impactful in delineating roles of certain neural groups in specific behavioural outputs. Under the optogenetic umbrella, channelrhodopsins are able to induce de novo neural action potentials or potentiate spiking [5] . However, this approach requires the delivery of light via a fibre-optic cable to the site where the opsins are expressed. These methods are not only invasive and cause tissue damage but may also hinder natural behaviour in some settings. To circumvent these problems, others have utilized engineered G s - or G q -protein coupled receptors, most notably, designer receptors exclusively activated by designer drug , which are activated by small compounds to potentiate electrically active cells [1] , [7] , [42] . Although this pharmacologically induced activation does not require direct access to the targeted cell group, the period between drug administration to peak activity and return to baseline is on the order of hours. Even though such long periods of induced activity have been beneficial in some experiments, this could confound interpretation of results in other settings [1] , [8] . More recently, a variety of chimeric ion channels have been generated that take advantage of the modular nature of Cys-loop receptors [10] . Although the inhibitory versions of these pharmacologically selective actuator modules have been demonstrated to be useful in vivo , the activators have not been fully tested in behaving animals and await further validation of their utility. STEMA fills a void between these tools by offering the following advantages. Similar to other small ligand-activated effector systems, the activation of TRPV1 can be achieved by systemic or oral administration of BBB-permeable capsaicin. This confers an appreciable advantage over systems that require the direct delivery of light or pharmacological agents to the site of action. Systemic application of capsaicin allows for activation of genetically identified diffuse central neurons as well as electrically active, non-neuronal peripheral targets like keratinocytes or pancreatic cells. Although temporal resolution of capsaicin-induced neural activation is far from the millisecond responses, its behavioural effects are faster than other small ligand-gated methods that peak in tens of minutes and last many hours (that is, designer receptors exclusively activated by designer drugs) [1] , [7] , [8] . The off-kinetics of STEMA provides an advantage in experiments that benefit from short neural-activation periods. Moreover, TRPV1 is directly coupled to neural electrical activity that circumvents potential problems caused by methods that require second messenger cascades [1] , [43] . In addition, STEMA does not require precise surgical manipulations, and large experimental cohorts can be generated with relative ease. One drawback of STEMA is the requirement to maintain mice on Trpv1 knockout background. Numerous groups have utilized mouse lines that lack functional TRPV1 to uncover the role of this channel [44] . Although these knockout mice are grossly indistinguishable from wild-type mice, they exhibit various peripheral deficits that range from inability to sense capsaicin to abnormal bladder control. The most prominent phenotypes, however, have been their impairment in noxious temperature detection and reduced inflammation-induced thermal hyperalgesia [17] , [45] . Some groups have demonstrated a potential role for TRPV1 in the central nervous system [46] , [47] , [48] . However, it is still controversial whether TRPV1 is expressed in the adult brain except for few discrete populations of neurons at low levels [49] . Another caveat for STEMA is the potential of capsaicin-independent TRPV1 activity from the ectopically expressed channels. This might stem from either ligand-independent baseline channel opening or endogenous TRPV1 ligands in the central nervous system (for example, anandamide, N-arachidonoyl-dopamine) [50] . Although we did not observe any obvious changes in the baseline firing pattern of DA cells from DAT–TRPV1 mice in slices or in vivo , we cannot rule out the possibility of subtle changes that interfere with cell physiology. Capsaicin-induced, TRPV1-dependent excitotoxicity has been described and observed in mice ectopically expressing TRPV1 in the striatum following local infusion of high dose (10 μM) but not lower doses (500 nM) of capsaicin [12] . Within the dose range of capsaicin used in this study, we did not detect obvious neural damage most likely due to the inability of peripherally administered capsaicin to reach sufficient concentrations in the brain. STEMA with its dose-dependent robust and rapidly reversible kinetics is a tractable, noninvasive effector system that will enrich our tool set of in vivo physiological and behavioural manipulations. The expansion of genetic driver lines and viral strategies that permit cell-type or connectivity-specific Cre recombinase expression will bolster the utility of STEMA in our pursuit of functional neural mapping. Furthermore, activation of TRPV1 with short pulses of infrared light or photoreleasable ligands could allow improved temporal resolution (for details on these potential technical advancements, see Supplementary Discussion ). STEMA and other effector systems will be instrumental in the decoding of the neural connectome and how it relates to physiology/behaviour in health and disease. Animals All experiments were conducted in accordance with approved animal protocols from the Institutional Animal Care and Use Committees of authors' institutions. All chemicals unless otherwise noted were purchased from Sigma. For i.p. capsaicin administrations, a stock solution was prepared at 3.2 mg ml −1 in vehicle (0.9% NaCl, 10% Tween-80) and sonicated until completely dissolved. Each dose was diluted using vehicle before use. Mice were house under 12-h light:dark cycle. Trpv1 knockout mice (B6.129X1- Trpv1 tm1Jul /J), obtained from The Jackson Laboratory, were crossed to Gt(ROSA)26Sor-stop flox -Trpv1-ires-ECFP , Slc6a3 Cre or ePet–Cre mice. These knockout lines were used to generate DAT–TRPV1 and ePet–TRPV1 mice. Female and male mice on a mixed 129Sv/C57BL/6J background (backcrossed to C57BL/6 for at least three generations) were used in all experiments. Except for slice electrophysiology (see below) mice were 2–5 months old during experimentation. Immunohistochemistry Primary antibodies to TH (monoclonal antibody 1:1,000, Chemicon), TPH (sheep antibody 1:1,000, Millipore), c-Fos (rabbit antibody 1:2,000, Calbiochem) and Iba1 (rabbit antibody 1:1,000, Wako) were used to detect immunoreactivity. Primary antibodies were detected using Cy2- or Cy3-conjugated, donkey anti-mouse or donkey anti-sheep and donkey anti-rabbit antibodies (1:300, Jackson Immunolabs). VTA slice preparations and electrophysiology Mice (postnatal day 25–35) were anaesthetized with halothane and killed. The brain was rapidly dissected, and horizontal slices (190-μm thick) containing the VTA were prepared using a Vibratome. Slices were allowed to recover for at least 45 min in artificial cerebrospinal fluid (containing the following (in mM): 126 NaCl, 3 KCl, 2.4 CaCl 2 , 1.2 NaH 2 PO 4 , 1.2 MgCl 2 , 18 NaHCO 3 , and 11 glucose, saturated with 95% O 2 and 5% CO 2 ) before being transferred individually to the recording chamber and superfused with continuous flow (2 ml min −1 ) of artificial cerebrospinal fluid at 32 °C containing picrotoxin (100 μM) to block GABA A receptor-mediated synaptic currents. Cells were visualized using an upright microscope with infrared illumination. Axopatch 1D amplifier (Axon Instruments) was used to perform whole-cell patch-clamp recordings with 2–6 MΩ electrodes. Dopamine neurons were identified by the pattern of spontaneous firing at 1–3 Hz, and the presence of hyperpolarization-activated current ( I h ) [51] . In voltage-clamp recordings, electrodes containing (in mM): 120 cesium methanesulfonic acid, 20 HEPES, 0.4 EGTA, 2.8 NaCl, 5 TEA-Cl, 2.5 MgATP, 0.25 MgGTP or 145 K-gluconate; 2 MgCl 2 ; 0.1 CaCl 2 ; 0.75 EGTA; 10 HEPES; 2 MgATP; 0.3 Na3GTP (at pH 7.2–7.4) were used to hold neurons at −70 mV. Capsaicin was applied for 8 min, after 8 min of stable recordings. Data were averaged in 2.5-min bins, normalized to baseline, defined as the average holding current of 30 consecutive sweeps before drug application, and presented as average across cells±s.e.m. For current-clamp recordings, 130 mM KOH, 105 mM methanesulfonic acid, 17 mM hydrochloric acid, 20 mM HEPES, 0.2 mM EGTA, 2.8 mM NaCl, 2.5 mg ml −1 MgATP, 0.25 mg ml −1 NaGTP (at pH 7.2–7.4 and 275–285 mOsm) internal solution was used. The firing activity was filtered at 2 kHz, digitized at 5–10 kHz, and analysed with Clampfit 8 software (Axon Instruments). After cell firing had stabilized, a baseline was recorded for 8 min and the mean firing frequency (in Hz) of each neuron was determined over the last 4 min, then CAP was applied for 5 min. Capsaicin effects were evaluated the 4 min spanning the last 2 min of its application and the first 2 min of wash out. Electrophysiology in freely moving mice HS-16 four-tetrode microdrives (Neuralynx) were implanted in anaesthetized mice by using stereotaxic coordinates for the VTA (−3.25 mm A-P, 0.5 mm M–L, and 4.5 mm D–V). After 2 weeks of recovery, mice were connected to a digital Lynx (10S) acquisition system through an HS-16 headstage preamplifier (Neuralynx), and signals were amplified and filtered (600–6000 Hz). Data were acquired by using Cheetah acquisition software (Neuralynx). Baseline putative DA neuron firing properties were recorded for 10 min, followed by 10-min post-capsaicin or vehicle i.p. administration period in an open-field. Tetrodes were lowered 50 μm daily during scanning for distinct units. Tetrode placement was confirmed post mortem by cresyl violet staining of 30-μm sections. Offline Sorter software (Plexon) cluster analysis was used to isolate units. Clustered waveforms were subsequently analysed with MATLAB (MathWorks). Baseline activity recordings (10 min) were used to identify putative DA neurons that exhibited broad (~2 ms), tri-phasic action potentials with firing rate <15 Hz. Standard score ( z score) is calculated as the difference of firing rate (spikes per second) within each 10-s bin from the mean baseline rate divided by the standard deviation during baseline. For peak firing rate and burst set rate (burst sets per second), spike activity was analysed in 2-min bins. A burst set was defined as an event initiated by 3 spikes with ≤80 ms inter-spike-interval and ended with an interval of ≥160 ms. Fast-scan cyclic voltammetry Mice were anaesthetized with urethane (1.5 g kg −1 ). A 150-μm diameter bipolar stimulating electrode (Plastics One) attached to an analog stimulus isolator (Iso-flex, AMPI), and a glass-encased, carbon-fibre microelectrode were placed at stereotaxic coordinates dorsal to MFB and NAc, respectively (for MFB: −2.4 mm A–P, 1.1 mm M–L; for NAc: 1.52 mm A–P, 1.15 mm M–L). Stimulation patterns were generated using Tarheel CV (National Instruments). The carbon-fibre was cycled at 60 Hz to allow the electrode to equilibrate and switched to 10 Hz for data acquisition. The stimulating and working electrodes were lowered in 150-μm increments until maximal DA release was observed (average D–V coordinates for MFB: 4.7 mm; for NAc: 3.86 mm). The average of four peak DA oxidation currents induced by MFB stimulations at 150 μA and 60 Hz for 1 s was calculated for each animal. For capsaicin-evoked responses, cyclic voltammograms were recorded at 10 Hz. Following a 2-min baseline, capsaicin was administered and responses were recorded for extra 33 min. Tarheel CV software was used for analysis of cyclic voltammograms. DAT–TRPV1 responses were aligned to initial detectable dopamine signal. Controls are aligned to DAT–TRPV1 mean detection time after capsaicin injection. Locomotion For monitoring distance travelled following drug administration (in DAT–TRPV1 experiments), mice were placed in 16×27 cm arena and video-recorded with a Canopus MediaCruise acquisition system for 30 min. Ethovision video analysis software (Noldus Information Technology) was used to track and calculate travelled distance. General activity was measured as consecutive beam breaks in activity chambers (San Diego Instruments). Before drug administration, animals were habituated for 2 h. Food consumption Food consumption by mice was measured using BioDAQ food monitoring system (Research Diets). Singly housed mice were placed in chambers and their daily chow (Research Diets D12450B) intake was recorded. After minimum of 4 days of habituation, access to food was blocked for 22 or 14 h at ZT 12. Before mice were allowed access again, they were administered capsaicin or vehicle. The latency to eat and the amount of food consumed were monitored via BioDAQ system. Two-bottle capsaicin preference Singly housed mice with two identical bottles were used to monitor amount of liquid consumed. Animals were acclimated to their chambers for 2 days with ad libidum food and normal water access. Natural capsaicin powder from hot chili peppers (containing 72% capsaicin and 24% dihydrocapsaicin by HPLC NutriScience Innovations) was used to prepare 0.325 g ml −1 stock solution in ethanol and mixed until dissolved. For pure capsaicin (97% by HPLC, Sigma) experiments, a 1-M stock solution was prepared in ethanol. These stock solutions were diluted 1,000-fold in 1% Tween-80 and 0.01% almond or vanilla flavouring to make capsaicin-containing drinking water. Control solution contained 0.1% ethanol, 1% Tween-80 and 0.01% almond or vanilla flavouring. For each chamber, one flavour was paired with capsaicin, the other with vehicle, and counter balanced to avoid flavouring preference. Vehicle and capsaicin solution consumption were monitored over 8 days to allow mice to associate one type of flavour with the effects of capsaicin. During this time, mice were allowed to access to only one of the two solutions per day and the locations of the solutions were switched daily to avoid side preference. After this association phase, animals were given free access to both of the solutions for 4 days. In this period, the locations of solutions were switched each day and consumption was monitored. During all phases of this experiment, animals had ad libidum access to normal chow. Open-field Following capsaicin administration, ePet–Cre or control mice were placed in a circular arena with a diameter of 48 cm and video-recorded with a Canopus MediaCruise acquisition system for 15 min. A virtual concentric circle with a diameter of 32 cm defined the centre zone. Ethovision video analysis software (Noldus Information Technology) was used to track and calculate travelled distance and time spent in each zone. Statistical analyses GraphPad Prism (GraphPad Software) was used for all statistical and nonlinear regression analyses. Repeated-measures or one-way ANOVA was used for multivariate analysis. Bonferroni or Tukey's post-tests were performed where appropriate. Student's t -tests were performed using two-tailed distribution. How to cite this article: Güler, A. D. et al . Transient activation of specific neurons in mice by selective expression of the capsaicin receptor. Nat. Commun. 3:746 doi: 10.1038/ncomms1749 (2012).